Proteasome assembly from 15S precursors involves major conformational changes and recycling of the Pba1–Pba2 chaperone The chaperones Ump1 and Pba1–Pba2 promote efficient biogenesis of 20S proteasome core particles from its subunits via 15S intermediates containing alpha and beta subunits, except beta7. Here we elucidate the structural role of these chaperones in late steps of core particle biogenesis using biochemical, electron microscopy, cross-linking and mass spectrometry analyses. In 15S precursor complexes, Ump1 is largely unstructured, lining the inner cavity of the complex along the interface between alpha and beta subunits. The alpha and beta subunits form loosely packed rings with a wider alpha ring opening than in the 20S core particle, allowing for the Pba1–Pba2 heterodimer to be partially embedded in the central alpha ring cavity. During biogenesis, the heterodimer is expelled from the alpha ring by a restructuring event that organizes the beta ring and leads to tightening of the alpha ring opening. In this way, the Pba1–Pba2 chaperone is recycled for a new round of proteasome assembly. The 26S proteasome is a 2.5-MDa protein complex tasked with timely degradation of polyubiquitylated proteins in eukaryotic cells. Proper function of the proteasome is vital to all eukaryotic life and malfunction has been implicated in a wide array of human diseases, including cancer and neurodegenerative disorders [1] , [2] . The 26S proteasome is composed of a barrel-shaped 20S core particle (CP) to the ends of which one or two 19S regulatory particles (RPs) are attached. While a high-resolution crystal structure of the eukaryotic 20S CP is known since 1997 (ref. 3 ), subnanometre structures of the 19S RP have only recently been determined by cryoelectron microscopy [4] , [5] , [6] . In eukaryotes, the 20S CP consists of seven distinctive alpha and seven distinct beta subunits, which are assembled into stacked rings, resulting in a characteristic α7/β7/β7/α7 architecture [3] . The β subunits form the proteolytic chamber, while the α subunits interact with regulatory complexes and promote gating of the 20S CP [7] . Proteasome biogenesis is an ordered process aided by several chaperones [8] , which are thought to promote productive and prevent promiscuous subunit interactions [9] , [10] , [11] , [12] . Early steps in the assembly of the 20S proteasome are supported by the heterodimeric chaperones Pba1–Pba2 and Pba3–Pba4 (refs 13 , 14 ), which promote correct assembly of the alpha ring. Formation of an intermediate containing a complete alpha ring and the β2, β3 and β4 subunits [15] , [16] requires displacement of Pba3–Pba4 (ref. 17 ). In yeast, the next detectable intermediate in the biogenesis pathway additionally contains the 17-kDa chaperone Ump1, β5, β6 and β1 (refs 16 ) and it is termed the 15S precursor complex (PC) based on its sedimentation properties in sucrose gradients [19] . Addition of the β7 subunits completes the assembly and leads to rapid dimerization of two half-proteasomes through intercalation of the C-terminal β7 extensions between β1 and β2 in the opposite beta ring [16] , [20] . Once the early 20S proteasome precursor is formed, autocatalytic pro-peptide cleavage of the proteolytic subunits β1, β2 and β5 takes place [21] . Upon activation of the proteolytic sites, the pro-peptides of β6 and β7 are processed [22] , and Ump1 is degraded as the first substrate of the nascent proteasome [19] . Work in mammalian cells suggested that subsequently also the Pba1–Pba2 chaperone is degraded by newly formed active CP [23] . Although Pba1 and Pba2 (also known as Poc1 and Poc2) are not essential for viability in Saccharomyces cerevisiae [13] , [16] , knockout or knockdown, respectively, of the mammalian orthologue of Pba1, termed PAC1, causes embryonic lethality in mice or severe defects in proteasome assembly in cultured human cells [23] , [24] . The two proteins form a stable heterodimer, which was reconstituted and crystallized with mature 20S CP from yeast [25] . In this structure, the C-terminal HbYX motif of Pba1 interacts with the intersubunit pocket between α5 and α6, which can also bind to the HbYX motif of Blm10 or of the 19S RP subunit Rpt5 (refs 7 , 26 , 27 ). Despite featuring a similar HbYX motif, Pba2 interacts in a different manner with the α6/α7 pocket making a smaller contribution to binding of the heterodimer [25] , [28] . The central channel, which is formed in the alpha ring of activated CP [29] , [30] , is closed in Pba1–Pba2-bound proteasomes [25] . Ump1 was the first chaperone found to be involved in proteasome biogenesis. Its deletion is not lethal in yeast, but makes cells hypersensitive to various forms of stress and leads to an accumulation of aberrant 20S CPs with unprocessed beta subunits [19] . The deletion of Ump1 can rescue lethality caused by deletions of the pro-peptides of either β5 or β6, pointing to a possible physical interaction between Ump1 and these pro-peptides [19] , [16] . Structural analyses have been reported for precursors of prokaryotic proteasomes, which assemble without dedicated chaperones [31] , [32] . No structures are available for precursors of the more complex eukaryotic CP bearing the above-mentioned chaperones Ump1 and Pba1–Pba2. Here we use single-particle electron microscopy (EM) combined with chemical cross-linking and mass spectrometric (CX-MS) analysis to investigate the subunit arrangement and chaperone localization in proteasomal precursors. Compared with the structure of a Pba1–Pba2–20S complex, we find substantial conformational changes within the alpha and beta rings of 15S PCs, with the Pba1–Pba2 heterodimer semiembedded in the centre of the alpha ring. Upon maturation of the 20S CP, the Pba1–Pba2 chaperone is ejected from the pore and recycled. Tracing the amino-acid chain of Ump1 in the 15S PC reveals interactions with multiple proteasomal alpha and beta subunits indicating an unstructured, extended conformation of this chaperone. Structure of the 15S proteasome PC The abundance of the 15S intermediate in the proteasome biogenesis pathway is very low in wild-type cells. In order to enrich the cellular 15S precursor population and to enable selective affinity purification, we used a yeast strain lacking the C-terminal extension of β7 (β7ΔCTE) [18] and expressing an N-terminally FLAG-6 × His (FH)-tagged version of Ump1. The β7ΔCTE mutation does not affect the structure of the 15S intermediate because the β7 subunit is absent from this complex [18] ; however, lack of the CTE causes an accumulation of the 15S PC because it inhibits 20S CP formation by complex dimerization [20] . We used a tagged version of Ump1 for a selective purification of the 15S PC because this assembly chaperone represents the only polypeptide that is associated with the 15S PC but not with 20S CPs. Initial affinity purifications of FH-tagged complexes from this strain not only yielded the 15S PC, but also many complexes lacking the Pba1–Pba2 chaperone, some of which were associated instead with Blm10 ( Fig. 1a ). To increase homogeneity of the precursor population, we introduced a deletion of the BLM10 gene and overexpressed the Pba1–Pba2 heterodimer. A strain with these modifications produced the 15S PC as the dominant proteasomal complex ( Fig. 1a,b ). The subunits of the purified PCs derived from this strain were separated by SDS–PAGE and subsequent peptide mass fingerprint analysis detected Pba1, Pba2, Ump1 and all 20S subunits but β7 ( Fig. 1c ). The identification of precursor forms of β2 and β5 in this preparation confirmed that the purified FH 15S complexes represent assembly intermediates ( Supplementary Fig. 1a ). These complexes were analyzed by negative stain EM and single-particle image-processing ( Fig. 1d , Supplementary Fig. 1b ). Multivariate statistical analysis of top view images did not reveal any heterogeneity caused by partial dissociation of Pba1–Pba2 in this data set ( Supplementary Fig. 1c ). Analysis of reference-free two-dimensional (2D) class averages revealed a sevenfold rotational symmetry in the top views of the complex and two-layered side views ( Fig. 1d ). The asymmetric three-dimensional (3D) reconstruction of the FH 15S complex has a diameter of 128 Å and a height of 112 Å ( Fig. 1e ). It shows a double ring structure with an internal diameter of ~30 Å, which is capped by a dimeric density on one side. The Pba1–Pba2 heterodimer and the alpha subunits fit the dimeric density and the seven equally strong densities underneath. Interestingly, we identify strong connecting density between the alpha ring and the beta ring for all but one alpha subunit, indicating that binding of the incoming beta subunits during FH 15S PC biogenesis involves interaction with their corresponding alpha subunits. The densities of the FH 15S PC beta ring are less well distinguishable, making it difficult to determine the exact positions of the six beta subunits and their propeptides ( Supplementary Fig. 1d ). The low resolution of the reconstruction (19.3 Å, Supplementary Fig. 1e ) and the ambiguous placement of the beta subunits preclude a precise localization of Ump1 in the EM map even at lower isosurface thresholds. As the FH 15S PC is purified via an N-terminal FH tag, this end of Ump1 appears to be easily accessible. We confirmed this notion by labelling FH–Ump1 with 5-nm Nanogold Ni 2+ NTA particles and subsequent negative stain analysis. Nanogold binding forces the FH 15S particles into side-view orientations ( Supplementary Fig. 2a ), suggesting that the N terminus of Ump1 is exposed at the beta ring opening because the alpha ring opening is occupied by Pba1–Pba2. A position of the Ump1 N terminus at the beta ring opening is, furthermore, consistent with the observation that an N-terminal green-fluorescent protein (GFP)–Ump1 fusion severely inhibited cell growth and 15S PC dimerization ( Supplementary Fig. 2b,c ). 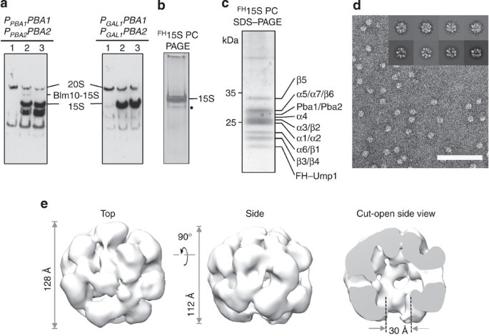Figure 1: Negative stain structure of the 15S proteasomal precursor (PC) complex. (a) Overexpression of Pba1–Pba2 increases the amounts of 15S PCs formed. Comparison of β2-containing complexes in wild-type cells (1), orFH-UMP1 PRE4-ΔCTEcells with (2) or withoutBLM10(3) by native PAGE analysis. Left panel, wild-type expression ofPBA1andPBA2. Right panel, overexpression ofPBA1andPBA2from PGAL1. (b) PurifiedFH15S complex analysed by native PAGE and silver staining. (c) Same as inb, but using 12% SDS–PAGE and Coomassie staining. Subunits of the complex were identified by peptide mass fingerprinting. (d) 15S PC micrograph with projections (inset, top row) and re-projections (inset, bottom row); scale bar, 100 nm; (e) 15S PC 3D reconstruction based on negative stain data. Figure 1: Negative stain structure of the 15S proteasomal precursor (PC) complex. ( a ) Overexpression of Pba1–Pba2 increases the amounts of 15S PCs formed. Comparison of β2-containing complexes in wild-type cells (1), or FH-UMP1 PRE4-ΔCTE cells with (2) or without BLM10 (3) by native PAGE analysis. Left panel, wild-type expression of PBA1 and PBA2 . Right panel, overexpression of PBA1 and PBA2 from P GAL1 . ( b ) Purified FH 15S complex analysed by native PAGE and silver staining. ( c ) Same as in b , but using 12% SDS–PAGE and Coomassie staining. Subunits of the complex were identified by peptide mass fingerprinting. ( d ) 15S PC micrograph with projections (inset, top row) and re-projections (inset, bottom row); scale bar, 100 nm; ( e ) 15S PC 3D reconstruction based on negative stain data. Full size image Ump1 cross-links to four proteasomal subunits We complemented the EM analysis of the FH 15S complex by CX-MS to independently verify the subunit arrangement and optimize our subunit fit into the EM density. Aside from the FH 15S PC used for the EM analysis, we also examined a 15S complex that carries a C-terminal GFP-HA tag on Ump1, but no N-terminal tag (15S GFP , Supplementary Fig. 3a ). Altogether, in the N- and C-terminally tagged complexes, we identified 52 and 56 distinct intersubunit cross-links, respectively ( Supplementary Tables 1–6 ). Out of these cross-links, 28 were found in both samples. The majority of intersubunit cross-links were found between alpha and beta subunits, confirming a subunit arrangement that is similar to that of the mature complex ( Fig. 2a , Supplementary Tables 1 and 2 ). Out of the 96 distinct intrasubunit cross-links in the FH 15S sample, we detected two cross-links (2.08%) that violated the maximum Cα–Cα cross-link distance of 30 Å ( Supplementary Table 3 ). 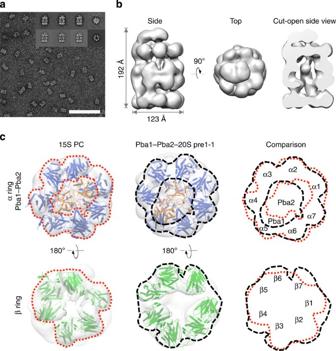Figure 3: Structural differences between the 15S and 20S complexes. (a) Micrograph of Pba1–Pba2–20Spre1-1sample with projections (inset, top row) and re-projections (inset, bottom row); scale bar, 100 nm; (b) Pba1–Pba2–20Spre1-13D reconstruction based on negative stain data. (c) Comparison between the subunit arrangement in the 15S precursor and the Pba1–Pba2–20Spre1-1complex. For a better overview, the α ring and Pba1–Pba2 (top row) are shown separately from the β ring (bottom row). The rate of unfit intrasubunit cross-links in the 15S GFP sample was at 5.21%, comprising the two unfit cross-links that are also found in the FH 15S sample plus three additional ones ( Supplementary Table 4 ). 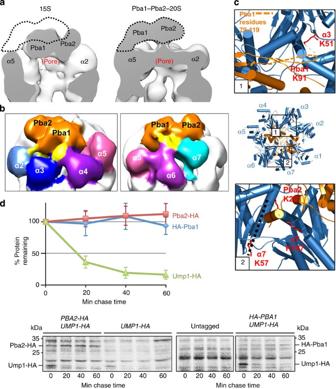Figure 4: Localization of Pba1–Pba2 in early and late proteasomal PCs. (a) Comparison between the positions of the Pba1–Pba2 heterodimer in the 15S precursor and Pba1–Pba2–20Spre1-1complexes seen as cut-open side view. A black dashed line outlines the position of the heterodimer in the Pba1–Pba2–20S pre1-1 complex. (b) Continuous EM density is formed between α subunits and the Pba1–Pba2 heterodimer in the 15S complex. EM densities corresponding to the individual subunits are coloured differently, with contact interfaces shown in yellow. (c) Cross-links found between the Pba1–Pba2 heterodimer and subunits α3 and α7. Lysine residues are shown as red sticks and cross-links are indicated by black dashed lines. The predicted loop region of Pba1 carrying K91 is shown as an orange dashed line. (d) Pulse chase assay to monitor turnover rates of HA-Pba1, Pba2-HA, and Ump1-HA, all expressed from their native promoters and genomic loci. The middle panel shows the nonspecific background signals obtained with radiolabelled proteins from an untagged control strain. The upper part shows the results of Phosphorimager quantification of HA-Pba1, Pba2-HA, and Ump1-HA signals. Error bars were calculated using the s.d. of four independent pulse chase experiments. Closer examination of all unfit cross-links reveals that each of them involves lysine residues located in loop regions of α1 (Lys58) or α4 (Lys53) or in a beta hairpin in β4 (Lys28). Thus, we omitted these regions when fitting the proteasomal subunits as rigid bodies into the EM density of the FH 15S PC. The fit was optimized manually so that subunits showed the smallest deviation from the mature complex, while simultaneously adhering to the EM map and the maximum Cα–Cα cross-link distance of 30 Å taking only intersubunit cross-links into account that were obtained in the CX-MS analysis of FH 15S PCs ( Fig. 2b,c ). Cross-links between non-neighbouring subunits were not taken into account, as they may have been formed arbitrarily (see below). Intriguingly, the CX-MS analysis shows that, apart from α7, all alpha subunits formed at least one cross-link to subunits of the beta ring. Thus, the lack of connecting density between one alpha subunit and the beta ring in the EM map is also reflected in the cross-linking profile of the complex. Most inter-ring cross-links appear between α1–α4 and β2–β4, indicating a higher structural integrity on this side of the half-barrel. 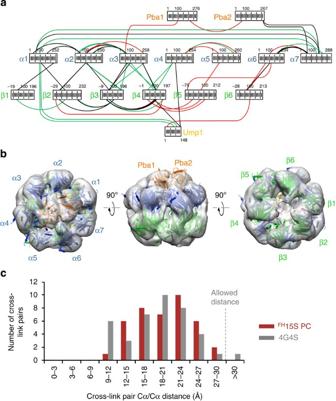This apparent feature of higher order on one side of the beta ring is also reflected in the EM map and fits previous descriptions on how the complex transitions from 13S to 15S precursor form (reviewed in refs 8 , 9 , 11 ). Together with the placement of the Pba1–Pba2 heterodimer in the alpha ring, it also allows us to unambiguously assign subunit densities in an otherwise pseudosymmetric complex. Figure 2: Cross-linking and MS analysis of the 15S complex. (a) Overview of intersubunit cross-linking data fromFH15S and 15SGFPcomplexes investigated by MS analysis. Subunits are shown as bars with the amino-acid numbering next to them. Lines indicate the cross-links. Cross-links shown in red were found inFH15S complexes, those in green in 15SGFPcomplexes and those in black in both complexes. GFP-related cross-links from the 15SGFPsample and cross-links that exceed the cross-link distance of 30 Å are not shown. (b) Proteasome subunits of the reconstituted Pba1–Pba2–20S complex (pdb: 4G4S) were fitted into the 15S EM map in accordance with restraints generated from cross-linking data and the EM map itself. The colour code is as follows: Pba1–Pba2 (orange), alpha1–7 (blue), beta1–6 (green) and 15S EM map (transparent grey). (c) Distances of 40 intersubunit cross-links obtained from theFH15S sample as shown inSupplementary Table 1were measured on the fit into theFH15S EM map (red) shown inFig. 3cand on the reconstituted Pba1–Pba2–20S complex (grey). Distances between Cα atoms of cross-linked lysines are measured. The maximum distance covered by DSS H12/D12 and two side chains of cross-linked lysines is ~30 Å. Figure 2: Cross-linking and MS analysis of the 15S complex. ( a ) Overview of intersubunit cross-linking data from FH 15S and 15S GFP complexes investigated by MS analysis. Subunits are shown as bars with the amino-acid numbering next to them. Lines indicate the cross-links. Cross-links shown in red were found in FH 15S complexes, those in green in 15S GFP complexes and those in black in both complexes. GFP-related cross-links from the 15S GFP sample and cross-links that exceed the cross-link distance of 30 Å are not shown. ( b ) Proteasome subunits of the reconstituted Pba1–Pba2–20S complex (pdb: 4G4S) were fitted into the 15S EM map in accordance with restraints generated from cross-linking data and the EM map itself. The colour code is as follows: Pba1–Pba2 (orange), alpha1–7 (blue), beta1–6 (green) and 15S EM map (transparent grey). ( c ) Distances of 40 intersubunit cross-links obtained from the FH 15S sample as shown in Supplementary Table 1 were measured on the fit into the FH 15S EM map (red) shown in Fig. 3c and on the reconstituted Pba1–Pba2–20S complex (grey). Distances between Cα atoms of cross-linked lysines are measured. The maximum distance covered by DSS H12/D12 and two side chains of cross-linked lysines is ~30 Å. Full size image In the 15S GFP sample, no intersubunit cross-links were detected for β5, and only one for β6, but intrasubunit and monocross-links confirm the presence of both subunits in this complex ( Supplementary Tables 4 and 5 ). In contrast, the FH 15S complex displays a larger number of cross-links for both subunits, indicating that the GFP moiety on the C terminus of Ump1 might alter the positioning of β5 and β6. Heterogeneity concerning the presence or absence of certain subunits was observed previously when the 15S GFP complex was purified via a Strep-tag on the C terminus of Ump1–GFP [33] . Cross-links involving the GFP moiety imply a flexible position of GFP inside the chamber formed by the alpha and beta rings ( Supplementary Table 6 ). Of particular importance are the cross-links involving the three chaperones. The CX-MS analysis of the FH 15S complex yielded seven intersubunit cross-links that involved Ump1, Pba1 or Pba2 ( Supplementary Table 1 ). Four of these cross-links were also found in the 15S GFP sample, two of which connect the C terminus of Pba2 to α7, while the other two connect the C terminus of Ump1 (K144) to α4 and β4, respectively. Thus, despite the possible re-arrangements caused by the C-terminal GFP tag in the 15S GFP complex, Ump1 seems to be incorporated correctly. Further cross-links between Ump1 and α1 (for 15S GFP ) or β6 (for FH 15S) suggest that the 17-kDa Ump1 protein stretches across the central cavity twice and is largely unfolded. Notably, cross-links between α1 and Ump1 are only observed in the 15S GFP complex. Nonetheless, we consider these cross-links valid as contacts between both proteins are also confirmed by two-hybrid data [34] . Altogether, three ( FH 15S) and five (15S GFP ) out of seven lysines of Ump1 formed cross-links or mono-links. All five intersubunit cross-links obtained from both samples involve Ump1 and lysines in helix 1 of alpha subunits or in helix 2 of beta subunits, all of which are located at the interface of the two rings. In the 15S GFP PC sample, one intraprotein cross-link is formed between the N-terminal and C-terminal segments of Ump1 in the 15S GFP complex. Thus, our data suggest that Ump1 loops along the inside surface of the α/β ring interface, interacting with four or more proteasomal subunits. In the final fit, all cross-links between neighbouring subunits in the FH 15S PC cover distances of 9–30 Å between the lysine Cα atoms ( Fig. 2c , Supplementary Table 1 ). In addition, ~10% of all intersubunit cross-links obtained in the FH 15S PC sample were found between non-neighbouring subunits, spanning distances of more than 30 Å ( Supplementary Table 1 ). All but one of these cross-links can be attributed to a distinct dimer between 15S complexes, which was found in the FH 15S PC sample in particular after cross-linking ( Supplementary Fig. 3b ). Similarly, two distinct dimers of 15S complexes can explain all cross-links between non-neighbouring subunits in the 15S GFP sample. 20S CP maturation involves re-arrangements of α and β rings In order for the 15S complex to adopt the 20S subunit arrangement, β7 needs to be incorporated into the structure, the beta subunits have to move into their final positions, the alpha ring pore needs to tighten up and the Pba1–Pba2 chaperone has to be either expelled or degraded. A reconstituted Pba1–Pba2–20S crystal structure indicates that the Pba chaperone binds to the CP in its closed gate conformation, probably precluding a degradation of the chaperones [25] . However, the crystal structure does not reflect a proteasomal assembly intermediate and Pba1–Pba2 might become enclosed and/or degraded by the maturing 20S CP during its assembly in vivo . We therefore investigated late precursor intermediates purified from a strain carrying a pre1-S142F ( pre1-1 ) mutation, which severely impairs proteasomal maturation in vivo leading to 20S CPs with enclosed Ump1 and associated Pba1–Pba2 ( Fig. 3a,b and Supplementary Fig. 3c ) [19] , [35] . The proteasome population isolated from extracts of this strain by affinity chromatography consisted mostly of mature proteasomes, but ~15% of the 20S pre1-1 proteasomes were still associated with one or two Pba1–Pba2 heterodimers ( Supplementary Fig. 3d ). An equal relative amount of proteasomal beta subunits was unprocessed in this population, suggesting that the Pba-containing proteasomes are late proteasomal precursors ( Supplementary Fig. 1a ). The 3D reconstruction of the Pba1–Pba2–20S pre1-1 complex from negative stain data at 21 Å resolution reveals a very similar subunit arrangement as seen for the reconstituted Pba1–Pba2–20S crystal structure, and we can dock the crystal structure as a rigid body into our EM map ( Supplementary Fig. 4a ). Figure 3: Structural differences between the 15S and 20S complexes. ( a ) Micrograph of Pba1–Pba2–20S pre1-1 sample with projections (inset, top row) and re-projections (inset, bottom row); scale bar, 100 nm; ( b ) Pba1–Pba2–20S pre1-1 3D reconstruction based on negative stain data. ( c ) Comparison between the subunit arrangement in the 15S precursor and the Pba1–Pba2–20S pre1-1 complex. For a better overview, the α ring and Pba1–Pba2 (top row) are shown separately from the β ring (bottom row). Full size image The subunit positioning in the FH 15S complex obtained by EM notably deviates from the arrangement in the Pba1–Pba2–20S pre1-1 complex ( Fig. 3c ). First, the Pba1–Pba2 densities are embedded in a cavity formed by the alpha ring, slightly pushing α5 and α6 outwards and rotating other subunits in order to create space in the central alpha ring opening. Second, the six subunits in the beta ring of the 15S PC are less ordered than in the heptameric beta rings of the 20S CP, which results in partial closure of the gap caused by the missing β7 subunit between β1 and β6. The poorly organized density of the beta ring in comparison with the alpha ring suggests that incoming beta subunits bind their corresponding alpha subunits, but do not occupy their final position until β7 incorporation or dimerization. Finally, our fit leaves some unfilled densities between β1 and β2 as well as β4 and β5, which are likely to correspond to the pro-peptides of the catalytic beta subunits, Ump1 or parts thereof. Pba1–Pba2 is expelled from the alpha ring during maturation In comparison with the Pba1–Pba2–20S pre1-1 complex, the EM map of the FH 15S PC reveals a strikingly closer association of Pba1–Pba2 with the rest of the complex ( Fig. 4a ). The alpha ring opening in the FH 15S complex is very wide with the Pba1–Pba2 heterodimer semi-embedded in a central position. In the EM map, continuous density exists between the heterodimer and all alpha subunits, except for α5. The strongest connections are observed near α3 and α4, as well as α6 and α7 ( Fig. 4b ). These interactions are not only seen in the EM map, but were also confirmed by cross-links between Pba1 K91 and α3 K51, as well as the Pba2 C terminus (K261) and α7 (K57 and K167; Fig. 4c ) in the FH 15S sample. K91 is located in a predicted loop region of Pba1, which was not resolved in the crystal structure; therefore, the exact architecture of this contact remains unclear. The strong interaction of the Pba2 C terminus with α7 suggests that the HbYX motif of Pba2 already engages with the α6/α7 pocket during early steps of proteasome maturation. We furthermore identified one cross-link between Pba1 K213 and Pba2 K65 in the FH 15S sample, verifying the layout of the heterodimer as seen in the crystal structure of the reconstituted complex. It is surprising that neither the EM map nor the cross-linking and MS analysis showed an interaction between Pba1 and the canonical α5/α6 HbYX-binding pocket. In fact, no cross-links were found between α5 and α6 either, and our fit of the crystal structures in the FH 15S EM map indicates a rotation of α5, which significantly alters the layout of the binding pocket. Figure 4: Localization of Pba1–Pba2 in early and late proteasomal PCs. ( a ) Comparison between the positions of the Pba1–Pba2 heterodimer in the 15S precursor and Pba1–Pba2–20S pre1-1 complexes seen as cut-open side view. A black dashed line outlines the position of the heterodimer in the Pba1–Pba2–20S pre1-1 complex. ( b ) Continuous EM density is formed between α subunits and the Pba1–Pba2 heterodimer in the 15S complex. EM densities corresponding to the individual subunits are coloured differently, with contact interfaces shown in yellow. ( c ) Cross-links found between the Pba1–Pba2 heterodimer and subunits α3 and α7. Lysine residues are shown as red sticks and cross-links are indicated by black dashed lines. The predicted loop region of Pba1 carrying K91 is shown as an orange dashed line. ( d ) Pulse chase assay to monitor turnover rates of HA-Pba1, Pba2-HA, and Ump1-HA, all expressed from their native promoters and genomic loci. The middle panel shows the nonspecific background signals obtained with radiolabelled proteins from an untagged control strain. The upper part shows the results of Phosphorimager quantification of HA-Pba1, Pba2-HA, and Ump1-HA signals. Error bars were calculated using the s.d. of four independent pulse chase experiments. Full size image In comparison with the arrangement of the FH 15S complex, the Pba1–Pba2 heterodimer is shifted out of the central cavity and moved towards α5 in the Pba1–Pba2–20S pre1-1 complex, giving the complex an asymmetric appearance. The alpha ring pore in the structure is closed. Continuous density between Pba1 and the α5/α6 interface indicates an HbYX-mediated binding mode of Pba1 in late PCs ( Supplementary Fig. 4b ). Interestingly, we also observe continuous EM density extending from Pba1–Pba2 to α3, but not from Pba2 to α7, suggesting that Pba1 and Pba2 have distinct roles during different stages of proteasome maturation. Our results indicate that yeast Pba1–Pba2, contrary to what had been concluded for its counterpart (PAC1–PAC2) in human cells [23] , is not degraded during 20S CP biogenesis but is expelled from the structure during maturation. This conclusion suggests that, in contrast to Ump1, which is degraded by nascent proteasomes, Pba1–Pba2 is recycled for possible engagement in multiple rounds of 20S CP biogenesis. This notion is consistent with our observation that Pba1–Pba2 becomes a limiting entity in 15S PC formation in the FH-Ump1 β7ΔCTE background ( Fig. 1a ). In this strain, due to the massive accumulation of PCs and poor 20S CP formation, very little recycling of Pba1–Pba2 is possible, precluding engagement in multiple assembly rounds. In support of the recycling nature of Pba1–Pba2, we found, using the pulse chase method and chromosomally tagged strains, that Pba1 and Pba2 are metabolically stable in contrast to Ump1, which is rapidly degraded in the same cells ( Fig. 4d ). Our analysis of the 15S PC from yeast provides novel insights into the structural progression of 20S CP biogenesis as well as the roles of the assembly chaperones Ump1 and Pba1–Pba2. A trajectory map shows that Ump1 loops around the inner chamber of the 15S PC, contacting subunits at the interface of the alpha and beta rings ( Fig. 5a ). Contacts to alpha subunits have previously been observed for yeast Ump1 (ref. 34 ) and its human orthologue [36] . The stretched out conformation of Ump1 and the lack of defined EM density along the projected path fit its description as an intrinsically unstructured protein with little secondary structure elements [37] , [38] . It also explains how Ump1 can be degraded by the nascent proteasome without dissolving its tertiary structure first. Earlier biochemical studies showed that Ump1 is inaccessible to polyclonal antibodies after dimerization of half-proteasomes and that apart from its N-terminal 5-kDa Ump1 is largely protected against trypsin digestion within the 15S PC [19] . The first 50 residues of human Ump1 were also shown to be dispensable for precursor binding, but were needed for proteasome maturation [39] . Our Nanogold labelling and cross-linking data indicate that a small fraction of the N terminus of Ump1 is projecting out of the 15S PC through the beta ring opening, but the Ump1 K16-β6 K91 cross-link obtained in the FH 15S sample does not suggest that large parts of Ump1 stick out of the half-proteasomes. In fact, addition of a bulky GFP moiety to the N terminus of yeast Ump1 blocks dimerization of the complex and inhibits cell growth ( Supplementary Fig. 2c ). The detected cross-link between Ump1 K16 and β6 K91 rather suggests that the N terminus of Ump1 is located near the interface of β6 and the incoming β7 subunit; therefore, it is possibly able to sense the arrival of β7 in the complex. The C-terminal half of Ump1 is required for binding to the proteasome, and cross-links to α4 and β4 found in both samples suggest that this part of Ump1 associates more tightly with proteasomal subunits than the rest of the protein. 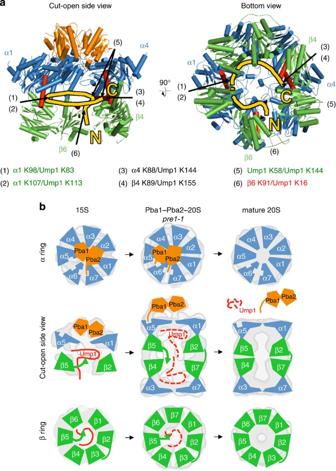Figure 5: Ump1 trajectory in the 15S PC and model of proteasome maturation. (a) Projected Ump1 trajectory in the 15S PC shown in a cut-open side view lacking α2/α3/β2/β3 (left) and bottom view lacking Pba1-Pba2 (right). Pba1–Pba2 is shown in orange, alpha subunits in blue and beta subunits in green. The projected Ump1 trajectory is shown as a yellow line. The N- and C termini are indicated. Cross-linking sites are indicated and marked by arrows. Cross-link description is colour-coded as follows: found only in 15SGFPsample, green; found only inFH15S sample, red; found in both samples, black. H1 or H2 helices in the cross-linking subunits are shown in red. (b) Maturation pathway from 15S precursor to the mature 20S complex. Schematic drawings of subunits show the subunit re-arrangements during maturation. Subunits are schematically drawn in front of silhouettes generated from the 15S and Pba1–Pba2–20Spre1-1EM maps as well as the low pass filtered crystal structure of the mature 20S proteasome (pdb: 1G0U, ref.29). The subunits are colour-coded as shown ina. Figure 5: Ump1 trajectory in the 15S PC and model of proteasome maturation. ( a ) Projected Ump1 trajectory in the 15S PC shown in a cut-open side view lacking α2/α3/β2/β3 (left) and bottom view lacking Pba1-Pba2 (right). Pba1–Pba2 is shown in orange, alpha subunits in blue and beta subunits in green. The projected Ump1 trajectory is shown as a yellow line. The N- and C termini are indicated. Cross-linking sites are indicated and marked by arrows. Cross-link description is colour-coded as follows: found only in 15S GFP sample, green; found only in FH 15S sample, red; found in both samples, black. H1 or H2 helices in the cross-linking subunits are shown in red. ( b ) Maturation pathway from 15S precursor to the mature 20S complex. Schematic drawings of subunits show the subunit re-arrangements during maturation. Subunits are schematically drawn in front of silhouettes generated from the 15S and Pba1–Pba2–20S pre1-1 EM maps as well as the low pass filtered crystal structure of the mature 20S proteasome (pdb: 1G0U, ref. 29 ). The subunits are colour-coded as shown in a . Full size image While the cross-linking data do not provide evidence of Ump1 interacting with the pro-peptide of β5, this interaction has been suggested by genetic data from yeast [19] and by biochemical data for its human orthologue hUMP1 (ref. 40 ). We observed cross-links between the β5 pro-peptide and α6 K115 in helix 2 in the FH 15S sample, which indicate close proximity between both segments. Thus, the β5 pro-peptide seems to cross the projected path of Ump1 somewhere along the N-terminal half of Ump1, permitting a direct interaction between Ump1 and pro-β5. The cross-link also suggests that the β5 pro-peptide is directed towards the alpha ring rather than pointing out of the cavity, arguing against a direct role of pro-β5 in dimerization of proteasome PCs at this stage of proteasome biogenesis, as previously discussed in ref. 16 . In the crystal structure of the reconstituted Pba1–Pba2–20S complex, the heterodimer is elevated above the alpha ring, mainly contacting the α5/α6 and α6/α7 pockets through its HbYX motifs [25] . In particular, the interaction between Pba1 and α6 features conserved contacts similar to those between proteasomal activators such as Blm10 or PA26 and the α5/α6 pocket. Intriguingly, our EM map and cross-linking analysis suggest a different binding mode of the heterodimer in the 15S PC. The embedded, central position of Pba1–Pba2, the increased pore diameter of the alpha ring and the connecting density to all alpha subunits, but α1 and α5, indicate that the heterodimer binds the N termini of the alpha subunits and displays a greater interaction area with the alpha ring than in late 20S PCs. Binding studies between archaeal components showed that PbaA requires the N-terminal 13 amino acids of the alpha subunit for interaction with 20S PCs [28] . Together with Pba3–Pba4, Pba1–Pba2 might indeed form a structural base, on which the alpha subunits assemble into a ring structure with the correct order during early proteasome biogenesis. Furthermore, we observe cross-links and connecting EM density in the FH 15S sample between Pba1–Pba2 and α3, the only nonessential subunit of the 20S proteasome. In the reconstituted Pba1–Pba2–20S complex, no connections between the chaperones and α1, α2 or α3 are made, raising the questions whether or how Pba1–Pba2 ensures correct incorporation of these three subunits in late proteasomal precursors. Our data suggest that large loop regions in the N-terminal region of Pba1 contact α3, possibly ensuring the alpha ring integrity once Pba3 and Pba4 are dissociated. In contrast to the mature proteasome and late PCs, the HbYX-binding pockets of the 15S precursors must be distorted because the subunits of the alpha ring create a large central opening. Notably, in the 15S PC, α6 is displaced towards α7, creating a greater distance between α5 and α6. This possibly prevents formation of a functional α5/α6 pocket and a canonical interaction with Pba1, but allows for an intact α6/α7 pocket and binding to Pba2. During precursor maturation, the alpha ring opening tightens and the subunits allocate to their final positions, forming the canonical HbYX-binding pockets. Tightening of the alpha and/or beta rings during maturation has previously been observed in proteasome PCs isolated from Archaeoglobus fulgidus [31] and Mycobacterium tuberculosis [32] , although the symmetry of those complexes, the lack of dedicated chaperones and the different nature of the beta subunit pro-peptides impede a comparison with the PCs presented in this study. In the Pba1–Pba2–20S pre1-1 complex, the binding mode of the Pba1–Pba2 chaperone resembles that seen in the reconstituted Pba1–Pba2–20S complex. After full maturation of the 20S, Pba1 and Pba2 are recycled for another round of proteasome maturation, indicating that their affinity to mature 20S proteasomes is lower than that to the PCs. Several studies already validated this hypothesis biochemically [16] , [23] , [28] , thereby also confirming the existence of changing binding modes of the Pba heterodimer during proteasomal biogenesis. On the basis of our analysis of CP PCs, we suggest that the Pba1–Pba2 heterodimer ensures correct assembly of the alpha ring in 15S complexes via its various interactions and keeps the subunits spread apart until the last beta subunit joins the PC ( Fig. 5b ). Incorporation of β7 into the beta ring not only establishes the layout of the beta ring, but also leads to a structural re-arrangement of the alpha ring possibly mediated by Ump1. As Ump1 is positioned ideally to sense β7 incorporation and convey this information to other regions of the half-proteasome via its multiple interactions, we agree with previous considerations [16] and suggest that Ump1 monitors the correct incorporation of subunits and prevents untimely dimerization of half-proteasomes. It possibly prevents the proteasomal subunits from prematurely locking into their final place, which would lead to expulsion of Pba1 and Pba2. Our data indicate that Pba1–Pba2 acts as a structural chaperone that is recycled after maturation, whereas the unstructured Ump1 possibly functions as a signal transducer rather than as a structural scaffold. Yeast media and strains Yeast rich (YPD) and synthetic (SD) minimal media with 2% dextrose were prepared as described [20] . Strain MO27 ( P GAL1 -PBA1::TRP1 P GAL1 - PBA2:HIS3 pre4-ΔCTE FH-UMP1 blm10 Δ ::KanMX6 ) was derived from AM31 (ref. 18 ) by successively inserting the P GAL1 promoter in front of the PBA1 and PBA2 genes using a PCR-based one-step gene transplacement strategy [41] . Strain MO29 ( ump1 Δ ::HIS3 PRE1-6His::YIPlac211/URA3 pre4 -Δ CTE::YIplac204/TRP1 with plasmid pMO2/ CEN-LEU2-P GALS -FLAG-GFP-UMP1 ) was derived from a JD281 spore clone (ML41-4C) [20] by generating the PRE1-6His allele using an integrative strategy and plasmid pJD315 (YIplac211-5′Δ pre1 - 6His -T CYC1 ), and subsequent transformation with pMO2. Strains MO23 ( pre1-1[S142F] [35] -FH ) and MO24 ( PRE1-FH ) were derived from the wild-type strain JD47-13C by a two-step gene transplacement strategy using plasmids pMO3 and pMO4, respectively. MO23 and MO24 were transformed with pJD657 ( CEN/URA3 P CUP1 -2xMYC-PBA1, PBA2, PBA3, PBA4-2xHA ). Strains with genomically tagged UMP1 and PBA2 (MO42 and MO43) were created by consecutively transforming, respectively, strains MO23 or MO24 with the integrative plasmids pJD490 ( UMP1-2HA ) and pFP2 ( PBA2-2HA ). Strain MK12 carrying a deletion of BLM10 and expressing Ump1 with GFP fused to the C terminus was created by transforming YIp5 Ump1-GFP-HA-TEV-ProA into BMF1 ( blm10Δ::HIS3 , ref. 42 ). Protein expression and purification The FH 15S complex was purified from a strain (MO27) grown in YP-galactose media, expressing FH–Ump1 and overexpressing Pba1 and Pba2. The F-GFP 15S complex was purified from a strain (MO29) expressing F-GFP Ump1 and Pre1 6H grown in selective minimal media with 2% galactose. Pba1–Pba2–20S pre1-1 complexes were purified from strain MO23 (with pJD657) grown in selective SD media with 100 μM CuSO 4 . Cells derived from these cultures were pelleted and frozen in liquid nitrogen. For preparation of the above-mentioned complexes, a tandem affinity purification protocol taking advantage of the FLAG and 6 × His tags was employed. The cells were ground to powder using a Mixer Mill MM400 (Retsch) for 1 min at 30 Hz. Proteins were extracted by incubating the powder with 2 ml g −1 wet weight FLAG buffer (50 mM Tris pH 7.5, 5 mM MgCl 2 , 2 mM ATP, 150 mM NaCl and 15% (v/v) glycerol, 10 mM imidazole with protease inhibitors (cOmplete, EDTA-free, Roche)) for 30 min at 4 °C with rotation. Cell debris was removed by centrifugation at 30,000 × g for 30 min at 4 °C, and the supernatant was passed through a 0.2-μm filter. The filtrate was incubated with 1.5 ml Ni 2+ sepharose resin equilibrated in FLAG buffer for 1 h at 4 °C with agitation. The resin was washed four times with 10 column bed volumes of FLAG buffer supplemented with 10 mM imidazole. Bound complexes were eluted in two steps with FLAG buffer supplemented with 50 and 100 mM imidazole. Eluted fractions were diluted 2.5 times in FLAG buffer and further incubated with anti-FLAG (M2) resin (Sigma-Aldrich) for 90 min at 4 °C with rotation. The beads were washed three times with 20 column volumes of FLAG buffer. Bound proteins were eluted with one column volume of FLAG buffer containing 0.3 mg ml −1 FLAG peptide (Sigma-Aldrich). Buffer was changed to either HEPES (25 mM HEPES, pH 7.5, 150 mM NaCl and 5% (v/v) glycerol) or FLAG buffer without glycerol and ATP by using NAP-25 Sephadex G-25 columns (GE Healthcare). Eluted material was then concentrated using Vivaspin 6 columns (50,000 MWCO, Sartorius Stedim Biotech). For preparation of the 15S GFP complex, MK12 yeast cells were grown in 3 L YPD at room temperature until an OD 600 of 3.0 was reached. Cells were harvested at 3,000 × g , followed by washing with ice-cold dH 2 O and buffer A (25 mM HEPES, pH 7.5, 150 mM NaCl, 1 mM EDTA, 5% (v/v) glycerol, 0.5 mM dithiothreitol). Pellets were re-suspended in buffer A supplemented with 0.002% (w/v) DNase I and one cOmplete protease inhibitor tablet. Lysis was performed using a FastPrep24 (MP Biomedicals). Cell debris was removed by centrifuging at 24,000 × g for 25 min at 4 °C. The cleared lysate was applied to IgG sepharose resin (GE Life Science) and incubated for 2 h at 4 °C. The column material was washed three times with 20 column volumes of buffer A and PCs were eluted by incubation with TEV protease for 2 h at room temperature. Purified complexes were analysed by native gel and/or SDS–PAGE as well as mass spectrometry (Central Bioanalytic Unit, Center of Molecular Medicine Cologne or Gene Center, LMU, Munich). Biochemical analysis of proteasome PCs Gel filtration, pulse chase analysis and SDS–PAGE were performed as described before [19] . Native PAGE utilized Ready Gels (Tris-HCl 4-15% gradient gels; Bio-Rad). Samples were mixed with NB4 × (240 mM Tris, pH 8.8, 80% (v/v) glycerol and 0.04% (w/v) bromophenol blue) and loaded onto the gel. Electrophoresis was performed in Laemmli running buffer without SDS at 16 mA for ~1.5 h with refrigeration. The gels were incubated for 10 min in transfer buffer containing 2% (w/v) SDS before electroblotting for 2 h at 0.8 mA cm −2 . Membrane processing and immunodetection were performed as described [19] . For pulse chase experiments, log-phase yeast cells were grown in the presence of 100 μCi [ 35 S]-methionine (10 mCi mmol −1 ) for 5 min, followed by a chase with cold methionine for 20, 40 or 60 min. Cell extracts prepared by glass bead in lysis buffer (50 mM Na Hepes, pH 7.5, 150 mM NaCl, 5 mM EDTA, 1% Triton-X100, 0.4% SDS and protease inhibitors (complete, Roche)) were subjected to immunoprecipitation with anti-HA resin (Sigma). After four washes with lysis buffer including 0.1% SDS, precipitated proteins were eluted by boiling in sample buffer, and analysed by SDS–PAGE, transferred to a nitrocellulose membrane and detected with a Typhoon FLA 7000 phosphor imager. Uncropped versions of all gel and blot scans used in the main and Supplementary Figs are presented in Supplementary Figs 5 and 6 . Chemical cross-linking and MS FH 15S and 15S GFP complexes were cross-linked with 0.8-mM disuccinimidyl suberate (DSS) H12/D12 (Creative Molecules) for 30 min at 30 °C before the reaction was quenched by adding ammonium bicarbonate to a final concentration of 100 mM. To further purify cross-linked 15S GFP complexes, they were spun through a 12-ml gradient consisting of buffer A and 10–40% (v/v) glycerol at 283,807 × g for 16 h. Fractions of the gradient containing 15S GFP complexes were concentrated using Amicon Ultra centrifugal filter units (100,000 MWCO, Millipore) and analysed by MS. FH 15S complexes were analysed by MS without additional purification by a glycerol gradient. The chemical cross-links on FH 15S and 15S GFP complexes were identified by MS analysis as described previously [43] . In short, cross-linked complexes were reduced with 5 mM tris(2-carboxyethyl)phosphine (Thermo Scientific) at 37 °C for 15 min and subsequently treated with 10 mM iodoacetamide (Sigma-Aldrich) for 30 min at room temperature in the dark. Digestion with lysyl enodpeptidase (Wako) at an enzyme–substrate ratio of 1–50 (w/w) at 37 °C for 2 h was followed by a second digestion with 1/50 (w/w) trypsin (Promega) at 37 °C overnight. Acidified peptides (1% (v/v) trifluoroacetic acid (TFA)) were purified by solid-phase extraction using C 18 cartridges (Sep-Pak, Waters). The eluate was dried by vacuum centrifugation and reconstituted in 20 μl of water/acetonitrile/TFA, 75:25:0.1. Peptides were separated on a Superdex Peptide PC 3.2/30 column (300 × 3.2 mm) at a flow rate of 50 μl min −1 . Fractions of 100 μl were collected and analysed by liquid chromatography coupled to tandem mass spectrometry using a hybrid LTQ Orbitrap Elite (Thermo Scientific) instrument. Fragment spectra were analysed using xQuest and the false discovery rate for both analyses was estimated below 3% using xProphet [44] . Electron microscopy Negative staining of proteasome PCs was performed using 2% (w/v) uranyl acetate. For screening of negatively stained grids, a Morgagni transmission electron microscope (FEI) equipped with an SIS Megaview 1-K charge-coupled device camera and running at 80 kV was used. Images were collected at a nominal magnification of × 60,000. For 3D reconstruction, micrographs were collected on a Tecnai G2 Spirit (FEI) and an Eagle CCD camera with 2,048 × 2,048 pixels. The pixel size was determined to be 2.9 Å at the specimen level using negatively stained 20S proteasomes for calibration. The microscope utilized a lanthanum hexaboride (LaB 6 ) electron source set to an extraction voltage of 120 kV. For imaging, the electron dose was set to 20 e − Å −2 . Images were collected at defoci between −0.3 and −1.0 μm. The contrast transfer functions were determined using CTFFIND3 (ref. 45 ) and phases were corrected for effects of the contrast transfer function in SPIDER [46] . Particles were either picked manually using EMAN1 boxer [47] or automatically using FindEM [48] . Particle stacks were subjected to sorting by XMIPP z -score [49] and false-positive particles were excluded based on visual inspection and class editing in IMAGIC [50] , yielding data sets of 10,156 particles for the FH 15S and 12,609 particles for the Pba1–Pba2–20S pre1-1 complex. After five rounds of classification based on multivariate statistical analysis followed by multireference alignment using homogenous classes as new references, eigen images of top view classifications of the FH 15S complex and of side view classifications of the Pba1–Pba2–20S pre1-1 complex, respectively, are analysed for significant peaks indicating heterogeneity in Pba1–Pba2 binding [51] . Initial 3D reconstructions of 15S and Pba1–Pba2–20S pre1-1 complexes were created using angular reconstitution in IMAGIC. For the 15S complex, initial 3D reconstruction employs C7 symmetry, which was relaxed to C1 symmetry after the first round of refinement. No symmetry was assumed during image processing of the Pba1–Pba2–20S pre1-1 data set. Euler angle assignment was refined using projection matching in SPIDER until >90% of the Euler angles were stable. Resolutions were determined using the FSC 0.5 criterion. Three-dimensional EM reconstructions were visualized using CHIMERA [52] and PYMOL (The PyMOL Molecular Graphics System, Version 1.5.0.4 Schrödinger, LLC). Contour levels of the isosurface representations were determined using chimera according to the expected molecular weight of the complexes, which are 431 kDa for FH 15S and 827 kDa for Pba1–Pba2–20S pre1-1 . How to cite this article: Kock, M. et al . Proteasome assembly from 15S precursors involves major conformational changes and recycling of the Pba1–Pba2 chaperone. Nat. Commun. 6:6123 doi: 10.1038/ncomms7123 (2015). Accession numbers: The 3D reconstructions of the 15S PC and the Pba1-Pba2-20S pre1-1 complex have been deposited in the EMBL-EBI EMDataBank under accession codes EMD-2656 and EMD-2658, respectively.